Correspondence: Reply to ‘Oncogenic MYC persistently upregulates the molecular clock component REV-ERBα’ Cell culture and transfections U2OS t-rex tetO-MYC cells [1] were maintained in DMEM supplemented with 10% FBS, 1x PenStrep, 50 μg ml −1 hygromycin, and 50 μg ml −1 zeocin (InvivoGen). All reagents for the cell culture were purchased from Life Technologies unless indicated differently. Twenty-four hours before synchronization, U2OS cells were transfected with siRNAs [1] using lipofectamine RNAiMAX reagent according to the manufacturer’s protocol. For luciferase recordings, U2OS cells were transfected with reporter constructs using Xfect (Clontech) and next day, cells were synchronized with 1 μM dexamethasone for 20 min and washed with PBS. After addition of warm luminescene medium (DMEM w/o Phenolred supplemented with 10% FBS, 25 mM Hepes, 1x PenStrep, and 0.125 μM luciferin (BioSynth), 10 ng ml −1 doxycycline) the plate was sealed and bioluminescence was recorded at 37 °C with an EnSpire Reader (Perkin Elmer). Gene expression analysis Total RNA was isolated using TriFaster (GeneON) and cDNA was synthesized with Maxima First Strand cDNA Synthesis Kit (Thermo Scientific). qPCR was performed using Green-Dye-Mastermix (Steinbrenner), TaqMan Gene Expression Master Mix (Applied Biosystems) and LightCycler 480 (Roche), and relative gene expression was quantified using a ΔΔCt method with respective reference gene ( GAPDH or B2M ). SYBR green primers were published previously [2] , [5] . 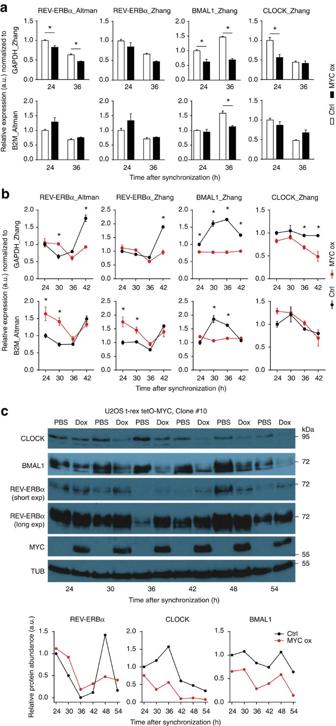Figure 1: Overexpression of MYC moderately increases REV-ERBα in U2OS cells. (a) qPCR reevaluation of RNA expression data from Shostaket al.1at two circadian time points using primers from Zhanget al.5and Altmanet al.2. Data were normalized toGAPDH(upper row) orB2M(lower row) by ΔΔCt (n=3). (b) qPCR analysis of circadian expression profiles of indicated transcripts in synchronized U2OS t-rex tetO-MYC cells normalized toGAPDH(upper row) orB2M(lower row) (n=3). qPCR products were detected with SYBR Green, corresponding quantification with TaqMan probes is shown inSupplementary Fig. 1a. (c) Western blot analysis (upper panel) and densitometric protein quantification (lower panel) of indicated proteins in synchronized U2OS t-rex tetO-MYC cells in presence (Dox) and absence (PBS) of overexpressed MYC (n=1). Data are presented as mean±s.e.m. *P<0.05; two-way ANOVA with Bonferroni post-test. 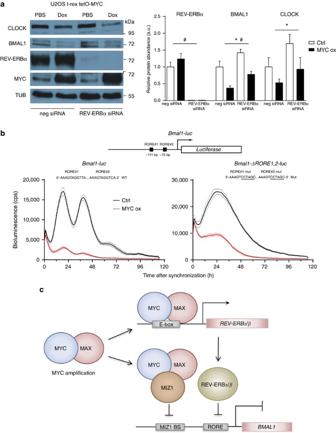Figure 2: MYC represses BMAL1 and CLOCK in absence of REV-ERBα. (a) MYC-dependent reduction of BMAL1 and CLOCK levels in presence and absence of REV-ERBα. U2OS t-rex tetO-MYC cells were transfected withREV-ERBαor negative siRNAs as indicated. After 24 h cells were treated with doxycycline to induce MYC (MYC ox) or with PBS for control (Ctrl). Western blot analysis (left) and densitometric protein quantification (right) (n=3) are shown. *P<0.05 for Ctrl versus MYC ox;#P<0.05 for neg siRNA versus REV-ERBα siRNA by two-way ANOVA. (b) MYC-dependent repression ofBmal1promoters with and without ROREs. Schematic of theBmal1-lucconstruct showing the location of ROREs. Sequence changes inactivating ROREs6,7are underlined (right panel). U2OS t-rex tetO-MYC cells transiently transfected withBmal1-luc(left) orBmal1-ΔRORE1,2-luc(right) were treated with doxycycline (MYC ox) or PBS (Ctrl) as indicated and, bioluminescence traces were recorded (n=3). Data are presented as mean±s.e.m. (c) Schematic of MYC-dependent direct and indirect repression of BMAL1. TaqMan primer sequences are listed in Supplementary Table 1 . Western blotting Protein lysates were prepared from synchronized U2OS t-rex tetO-MYC cells and blotted on nitrocellulose membranes. Membranes were incubated in 5% milk TBS at 4 °C overnight supplemented with anti-BMAL1 (ref. 1 ) (1:750), anti-CLOCK (ref. 1 ) (1:500), anti-Tubulin (1:1,000, WA3), anti-MYC (1:400, N-262, SantaCruz) and anti-REV-ERBα (1:1,000, 13418S, Cell Signaling) antibodies. Proteins were quantified using ImageJ by normalizing to Tubulin. Uncropped blots are shown in Supplementary Fig. 2 . Data availability The data supporting the findings of this study are available within the article and its Supplementary Information files, or from the authors on request. How to cite this article: Shostak, A. et al . Correspondence: Reply to ‘Oncogenic MYC persistently upregulates the molecular clock component REV-ERBα’. Nat. Commun. 8, 14918 doi: 10.1038/ncomms14918 (2017). Publisher’s note : Springer Nature remains neutral with regard to jurisdictional claims in published maps and institutional affiliations.